Atomic scale dynamics of ultrasmall germanium clusters Starting from the gas phase, small clusters can be produced and deposited with huge flexibility with regard to composition, materials choice and cluster size. Despite many advances in experimental characterization, a detailed morphology of such clusters is still lacking. Here we present an atomic scale observation as well as the dynamical behaviour of ultrasmall germanium clusters. Using quantitative scanning transmission electron microscopy in combination with ab initio calculations, we are able to characterize the transition between different equilibrium geometries of a germanium cluster consisting of less than 25 atoms. Seven-membered rings, trigonal prisms and some smaller subunits are identified as possible building blocks that stabilize the structure. Ultrasmall clusters have attracted increasing interest, because they can be thought of as fundamental building blocks leading to metamaterials with physical and chemical properties that are not available in nature [1] , [2] . Consequently, the structure of clusters of Ge and other group IV elements has been the subject of many studies. Whereas bulk Ge has the diamond cubic structure, the hitherto-identified structural growth mechanisms for small clusters are much more exotic. Early mass spectrometry observations of species with enhanced stability and fragmentation mass spectrometry have confirmed the existence of small-sized building blocks, in particular Ge 6-11 , with the most stable sizes being Ge 6 , Ge 7 and Ge 10 (refs 3 , 4 ). First structural assignments were based on ion-mobility experiments in combination with density functional theory computations [5] . Meanwhile, more extensive theoretical studies have revealed structural patterns consistent with stable deltahedral subunits where larger species consist of several of these subunits joined together forming, for example, prolate [6] (sizes N~30) and platelet [7] (sizes N~45) -shaped nanoparticles. Recent advances in the field of transmission electron microscopy (TEM) enable one to obtain two-dimensional (2D) images with a spatial resolution of up to 50 pm. However, it is still not straightforward to determine the three-dimensional (3D) geometry of ultrasmall clusters. One of the problems is that during electron irradiation, clusters may rotate or show structural changes [8] , [9] . Even though TEM observations can now be made at lower acceleration voltages or while cooling the sample, still, an intrinsic energy transfer from the impinging electron beam to the sample cannot be fully avoided. This results in the unique possibility to visualize the transformation between energetically excited configurations. Furthermore, the support on which the clusters are deposited may have a strong influence on their structure and dynamics. Here we determine different equilibrium configurations of ultrasmall Ge clusters deposited on a carbon support using state-of-the-art aberration-corrected TEM. Using statistical parameter estimation theory and ab initio calculations, we are able to analyse several metastable configurations that are reproduced as local energy minima. The direct observation of the atomic scale dynamics evidences a 2D-to-3D transition, as well as a transition from a compact towards an elongated structure of the cluster, which finally breaks up into smaller fragments. Quantitative 2D electron microscopy As explained in the Methods, ultrasmall Ge clusters preformed in the gas phase were deposited on TEM grids coated by a thin layer of amorphous carbon. The clusters are imaged using high-angle annular dark field scanning transmission electron microscopy (HAADF-STEM) at 120 kV. Under the electron beam, structural changes of the clusters are observed and the movement of single Ge atoms on the carbon support can be followed. The cluster shown in Fig. 1 was imaged by acquiring 100 frames with an individual frame time of 0.1 s. A subseries of eight consecutive frames ( Fig. 1a–h ) is studied here in more detail. Another example of a series of images is presented as Supplementary Fig. S1 . The configuration of the cluster in Fig. 1a appears predominantly 2D, whereas the configurations in Fig. 1g,h are observed with enhanced contrast at certain atom positions, suggesting a 3D geometry. To study this transformation, Fig. 1a , Fig. 1h and an intermediate frame ( Fig. 1d ) have been quantified by statistical parameter estimation theory [10] , [11] , [12] . Using this approach, a parametric model in which the projection of an atom corresponds to a Gaussian peaked at the atom position has been assumed. The parameters of this model, including the atom positions, the height and width of the intensity peaks, have been determined using the least squares estimator. The refined models, evaluated at these estimated parameters, are shown in Fig. 2a–c . From the estimated parameters, also totally scattered atom intensities, corresponding to volumes under the estimated Gaussian peaks, are determined. 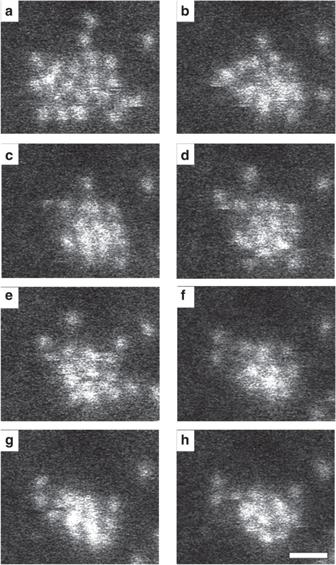Figure 1: Sequence of HAADF-STEM images of a Ge cluster. (a–h) Each subsequent image is acquired with a frame time of 0.1 s. It can be seen that a 2D-like configuration transforms into a 3D configuration. The scale bar corresponds to 0.5 nm. Figure 1: Sequence of HAADF-STEM images of a Ge cluster. ( a–h ) Each subsequent image is acquired with a frame time of 0.1 s. It can be seen that a 2D-like configuration transforms into a 3D configuration. The scale bar corresponds to 0.5 nm. 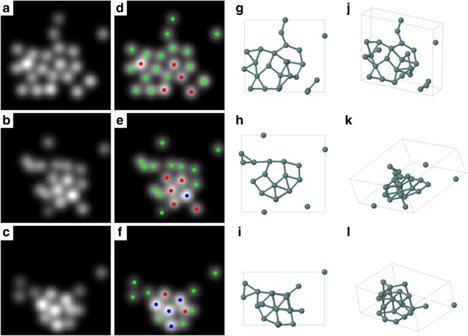Figure 2: 3D models derived from 2D experimental images. (a–c) Parametric models refined on the basis of the experimentalFig. 1a,d,h. (d–f) Counting results in which green, red and blue dots correspond to 1, 2 and 3 atoms, respectively. (g–l) Outcome of theab initiocalculations shown along two different viewing directions. Full size image Figure 2: 3D models derived from 2D experimental images. ( a–c ) Parametric models refined on the basis of the experimental Fig. 1a,d,h . ( d–f ) Counting results in which green, red and blue dots correspond to 1, 2 and 3 atoms, respectively. ( g–l ) Outcome of the ab initio calculations shown along two different viewing directions. Full size image HAADF-STEM intensities scale with the atomic number Z of the atoms present in a sample as well as with the number of atoms. Here all atoms are of the same type and, consequently, the intensity will increase when several atoms are positioned on top of each other. On the basis of such quantitative analysis, we conclude that the estimated peaks correspond to 1, 2 or 3 atoms projected on top of each other. These results are indicated in Fig. 2d–f and confirm that 2D, 3D and intermediate configurations are present. 3D structure characterization To evaluate the stability of these configurations, ab initio calculations have been carried out. The x and y coordinates in the starting configuration are directly based on our experimental results ( Fig. 2d–f ). Along the z direction, we assumed three equally spaced planes that may contain atoms as a starting point. We built up the 3D structure from the 2D projections based on a planar base structure on top of which additional atoms are added (in case of the presence of 2 or 3 atoms at the same 2D-projected position). After full relaxation, the Ge cluster geometries ( Fig. 2g–l ) stayed close to the initial configuration, demonstrating that they indeed correspond to local energy minima and that the measured clusters are stable. Of course, these planar base structures are not the only 3D structures compatible with the 2D experimental projections. Therefore, also other configurations were constructed as starting points for the ab initio relaxation, in which stacked atoms were moved over half or a full bond length. Two examples are presented in Fig. 3 . These configurations are still compatible with the 2D observations. However, after relaxation, it was found that these geometries showed a clear deviation from the experimentally observed images. In this way, the combination of 2D experimental images, statistical parameter estimation theory, and 3D density functional theory calculations allowed us to characterize the 3D geometry of the observed Ge clusters reliably. It must be noted that in our calculations, the amorphous carbon substrate was not taken into account as its exact structure is not known. However, recent calculations show that Ge physisorbs on graphane with a binding energy around 0.5 eV per Ge atom [13] . Therefore, we can conclude that the substrate stabilizes the clusters further. Moreover, from all possible local minima configurations, it can be expected that the substrate favours most of those clusters for which this stabilizing effect is maximal, that is, for geometries with a planar base structure. This is indeed supported by our analysis as described above. 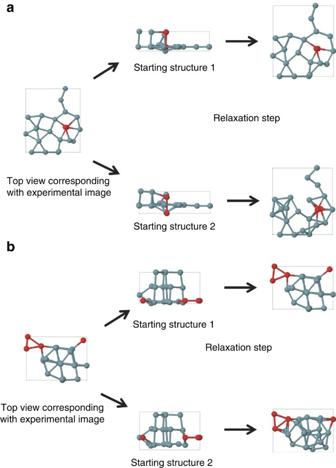Figure 3: Two examples of slightly varying starting configurations resulting in significantly altered relaxed structures. (a,b) The left panels represent the top view of a model that corresponds to the experimental picture. The panels in the middle give two different configurations that are indistinguishable if viewed from the top. After relaxation with density functional theory (panels on the right), only one of the two possibilities is still compatible with the experimental image, as can be seen inFigure 2. Figure 3: Two examples of slightly varying starting configurations resulting in significantly altered relaxed structures. ( a , b ) The left panels represent the top view of a model that corresponds to the experimental picture. The panels in the middle give two different configurations that are indistinguishable if viewed from the top. After relaxation with density functional theory (panels on the right), only one of the two possibilities is still compatible with the experimental image, as can be seen in Figure 2 . Full size image Cluster dynamics The number of atoms that form the cluster also changes. Although it is not straightforward to define the cluster size, we feel that it is reasonable to define the cluster size as being the sum of all atoms that are connected by bonds. To account for small variations in bond length, the maximum allowed distance to consider two Ge atoms as bonded was set to 1.2 times the average bond length. With this definition, the cluster sizes in Fig. 2 are 22 for the top row, 20 for the middle row, and 23 for the bottom row. For the 2D configuration, a binding energy per atom of −4.51 eV is found, whereas the 3D configuration has a binding energy of −4.64 eV per atom. Remarkably, the intermediate configuration corresponds to a less stable structure with a binding energy of −4.49 eV per atom. To study the transformation from the 2D configuration to the 3D configuration, we followed the path of each individual atom. Many possibilities exist, but it is a reasonable assumption that the most likely pathway is close to the shortest travelled distance of all atoms. Therefore, the total travelled distance has been minimized over all possible combinations of atoms in two successive frames. The results are presented in Supplementary Fig. S2 . In addition to the analysed configurations shown in Fig. 2 , several other configurations of the same cluster have been investigated using the same quantitative approach. One of these configurations, which appears after longer observation, is presented in Fig. 4 . The refined model evaluated at the estimated parameters is shown in Fig. 4a , whereas the result of the ab initio calculations is presented in Fig. 4b . This shows that the cluster has evolved from compact geometries to an almost planar strongly elongated shape. Also this structure was reproduced by the ab initio calculations with an average binding energy per atom of −4.24 eV. In this configuration, it is clear that the cluster is built up from smaller subunits very similar to the predicted configurations for clusters consisting of 3 and 4 atoms. Later observed frames show that the cluster breaks up into smaller fragments of 3–7 atoms. 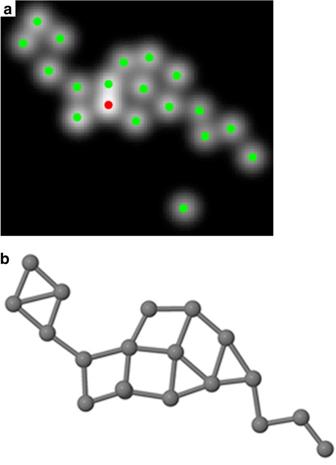Figure 4: Quantitative analysis of a more elongated prolate configuration. (a) Refined parametric model, peaked at the estimated atomic positions. Green and red dots correspond to 1 atom and 2 atoms, respectively. (b) Outcome of theab initiocalculation. It can be seen that a seven-membered ring is present. In addition, smaller fragments, consisting of 3–4 atoms are found to correspond well to the predicted ground states of trimers and tetramers. Figure 4: Quantitative analysis of a more elongated prolate configuration. ( a ) Refined parametric model, peaked at the estimated atomic positions. Green and red dots correspond to 1 atom and 2 atoms, respectively. ( b ) Outcome of the ab initio calculation. It can be seen that a seven-membered ring is present. In addition, smaller fragments, consisting of 3–4 atoms are found to correspond well to the predicted ground states of trimers and tetramers. Full size image In this study, we observe the transition between a 2D and a 3D configuration of a Ge cluster consisting of about 25 atoms. Structural re-arrangements such as the ones observed here were still present when cooling the sample to liquid nitrogen temperatures. In addition, according to Hobbs [14] , specimen heating is negligible for our specific sample and the beam current that was used. It is therefore likely that the main driving mechanism for the re-arrangements is knock-on momentum transfer [15] . The transferred kinetic energy is maximal for head-on collisions and depends on the ratio of the electron mass and the mass of the nuclei, as well as the acceleration voltage of the TEM. For Ge clusters imaged using an acceleration voltage of 120 kV, atom displacements in bulk Ge are not expected. However, sputtering of surface atoms and therefore displacements of the individual atoms in an ultrasmall Ge cluster are likely [16] . During our TEM investigations, bonds will therefore break and form at the timescale observed here. By comparison of the calculated binding energies, we conclude that the transition occurs between two low-energy metastable states through an intermediate higher energy state. The pathway from the 2D to 3D configurations includes the formation of regular trigonal prisms, which nicely corresponds to the theoretical prediction of (capped) trigonal prisms as structural motives in the development of elongated free-standing Ge clusters in this size range [17] . It is striking that both in the 2D and the 3D configurations shown in Fig. 2, as well as the elongated structure presented in Fig. 4 , seven-membered rings are present. Although we expect that the presence of a support will have a large influence on the formation of planar rings, it must be noted that, during the relaxation of the ab initio calculations, this planar structure was also observed to be stable in free space. It is therefore plausible that seven-membered Ge rings form stabilizing building blocks in larger 2D and 3D configurations with a planar base structure. The configuration in Fig. 4 shows the presence of smaller building blocks that correspond well to the configurations of Ge trimers and tetramers in their ground state [18] . After observation of this configuration, the cluster was found to break up into smaller fragments consisting of 3–7 atoms. Such fragmentation process was observed also in laser photofragmentation studies and ab initio calculations demonstrating that semiconductor clusters such as Si and Ge dissociate into fragments with a preference for 7–10 atoms [4] , [19] . In conclusion, we present a quantitative interpretation of the dynamical behaviour of ultrasmall semiconductor clusters. The dynamics of the cluster supported on a thin carbon layer can be followed atom by atom yielding unique insight concerning the stability of different building blocks including trigonal prisms and seven-membered rings, and the dynamical transition between these configurations. Our results furthermore show that 2D as well as 3D configurations with a planar base structure are stable. Cluster production and deposition Gas phase clusters were produced using a cluster source based on laser vapourization of a Ge target and condensation and aggregation in pulses of He carrier gas [20] , [21] . The cluster source is integrated in an ultrahigh vacuum cluster deposition chamber that is described in detail by Vandamme et al . [22] The size distribution of the clusters in the beam is monitored by time-of-flight mass spectrometry, showing clusters from the monomer to about 150 atom clusters. A mass spectrum of the cationic Ge clusters is shown in Fig. 5a . The cluster-size distribution was optimized for small sizes by reduction of the cluster source volume and by operating the source at room temperature, resulting in abundant production of species from Ge 6 up to about Ge 45 . Depending on the cluster shape, this corresponds to a diameter up to 17 Å for a planar disk or 13 Å for a sphere. Assuming a circular disk shape for the most abundant cluster, Ge 10 , a diameter of 9 Å is found. It should be noted, however, that larger clusters also may be present in the cluster beam but will not be registered because of a decreasing detector efficiency with cluster mass. 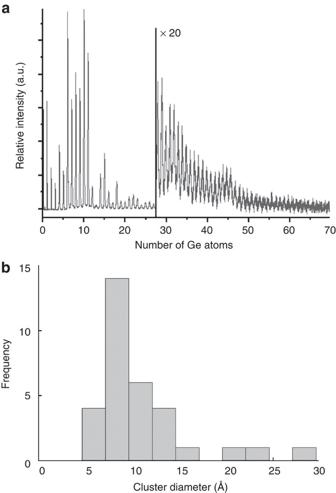Figure 5: Size distribution of the clusters. (a) Time-of-flight mass abundance spectrum of Ge cluster cations. Of interest are the strong size-dependent features reflecting enhanced stability for a number of sizes in the 6 to 20 atoms range. (b) Histogram illustrating the size distribution of the investigated clusters as deduced from the TEM images. It must be noted that, although this histogram contains only clusters with a diameter <2 nm, larger clusters (with sizes up to 10 nm) also have been observed. Figure 5: Size distribution of the clusters. ( a ) Time-of-flight mass abundance spectrum of Ge cluster cations. Of interest are the strong size-dependent features reflecting enhanced stability for a number of sizes in the 6 to 20 atoms range. ( b ) Histogram illustrating the size distribution of the investigated clusters as deduced from the TEM images. It must be noted that, although this histogram contains only clusters with a diameter <2 nm, larger clusters (with sizes up to 10 nm) also have been observed. Full size image The resulting beam of Ge clusters is subsequently deposited without size selection at room temperature on TEM grids, which consist of an ultrathin amorphous carbon layer supported by a Cu grid. The clusters were deposited with their inherent low kinetic energy (~0.15 eV per atom). This corresponds to a soft-landing regime, where the kinetic energy is small compared with the atomic binding energy within the cluster, and, consequently, negligible cluster fragmentation is expected owing to the impact [23] . Deposition times were chosen to achieve a low cluster density, well below complete coverage of the substrate. A histogram of the size distribution of all clusters as imaged by TEM is presented in Fig. 5b . As the clusters change their geometry during the TEM investigation, it is not straightforward to define the diameter. The diameter was measured for each cluster being in its most spherical, compact geometry. It must be noted that, although this histogram contains only clusters with a diameter <2 nm, larger clusters (with sizes up to 10 nm) also have been observed. The distribution corresponds well with the size distribution as registered during cluster production, indicating very limited cluster mobility and absence of coagulation upon landing on the substrate. TEM imaging The clusters have been imaged using HAADF-STEM performed using a double aberration-corrected FEI TITAN operated at 120 kV. Further experiments have been carried out at an acceleration voltage of 300 kV in combination with cooling of the sample at liquid nitrogen temperature. In addition, we have also explored the possibilities of cooling the sample at 80 kV and 120 kV. However, the ultrathin carbon support on the Cu grid was then observed to be unstable. Therefore, the final experiments were performed at 120 kV without further cooling of the sample. The beam current was set to 40 pA. Structural changes of the clusters have been observed in all experiments for clusters with a diameter smaller than 1 nm. A frame time of 0.1 s was used to image the clusters. Lower frame times will lead to a decrease of signal-to-noise ratio. The time resolution in our experiments can therefore be considered to be 0.1 s. Statistical parameter estimation The totally scattered atom intensities estimated by fitting a parametric model to the experimental images are influenced by several factors, including experimental detection noise and the dynamical character of the frames. As a consequence, quantifying the observed intensities, in terms of number of atoms, should be done in a statistical manner [10] . 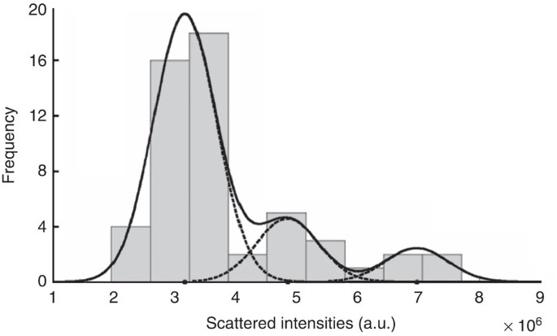Figure 6: Histogram of the totally scattered intensities. These intensities are determined from the estimated Gaussian peaks inFig. 2a–c. The solid curve shows the estimated mixture model; the individual components are shown as dashed curves. Figure 6, therefore, presents the histogram of all intensities corresponding to the estimated Gaussian peaks shown in Fig. 2 . Next, these intensities are regarded as independent statistical draws from a so-called Gaussian mixture model. This model, defined as a superposition of Gaussians, describes the probability that a specific intensity value will be observed. To determine the number of significant peaks of this model, the integrated classification likelihood criterion [10] , [24] was used, indicating the presence of three peaks. Their positions, amplitudes and width have been estimated using the so-called expectation maximization algorithm. Its aim is to optimize the likelihood that the given intensities are generated by a mixture of Gaussians. The solid curve in Fig. 6 shows the estimated mixture model; the individual Gaussian components are shown by means of dashed curves. Because of the inherent statistical measurement errors as described above, overlap of the Gaussian components is observed in Fig. 6 causing uncertainties for the number of atoms in specific Gaussian peaks. However, by exploiting the boundary conditions determined by the conservation of the total number of atoms in the area of interest, a unique solution for the number of atoms at each estimated position has been found. Figure 6: Histogram of the totally scattered intensities. These intensities are determined from the estimated Gaussian peaks in Fig. 2a–c . The solid curve shows the estimated mixture model; the individual components are shown as dashed curves. Full size image Ab initio calculations All calculations are based on density functional theory and performed using the OpenMX code [25] , [26] with periodic boundary conditions. We use the local density approximation functional developed by Ceperly and Alder [27] to evaluate the exchange-correlation energy of interacting electrons. Double-valence plus single-polarization orbitals are used as the basis set. A large enough vacuum space is used to treat the Ge clusters as isolated from each other. The relaxed structures have been optimized carefully without any constraint (that is, without forcing the clusters to form planar structures). The optimization, implemented in the OpenMX code, was based on the method described by Baker [28] . Starting configurations were based on the experimental measurements as shown in the first and second column of Fig. 2 . For the optimized structure calculations, all atoms in the system are relaxed until the forces are less than 0.005 eV/Å. How to cite this article: Bals, S. et al . Atomic scale dynamics of ultrasmall germanium clusters. Nat. Commun. 3:897 doi: 10.1038/ncomms1887 (2012).